Controllable unzipping for intramolecular junctions of graphene nanoribbons and single-walled carbon nanotubes Graphene, a two-dimensional (2D) single-atom thick crystal with carbon atoms arranged in a honeycomb lattice, has only been intensively researched since 2004. Nevertheless, it has attracted enormous interest from both theoretical and experimental scientists due to its monoatomic thickness, excellent properties and potential widespread applications [1] , [2] . As a candidate for future electronics, pristine graphene suffers from being a zero bandgap semiconductor. Hence, for practical applications, various modifications of graphene are required, which may allow graphene to be used as different components in future electronics [2] , [3] . The formation of graphene junctions with other materials can improve the properties of pristine graphene, allowing for its use in new device applications [4] . In this field, some pioneering theoretical studies have been performed [5] , [6] , [7] . However, it remains a challenge to fabricate these nanostructures, and much experimental effort is still needed to realize their practical applications. Carbon nanotubes (CNTs) and graphene are two carbon allostropes that have generated intense interest in the field of nanoscience; however, there have been few attempts to merge them at the molecular scale. Theorists have predicted novel properties intrinsic to the CNT–graphene intramolecular junction [5] , [6] , [7] , and experiments have also occasionally observed these junction nanostructures in unzipped CNT samples [8] . Here, we develop a sputter-etching method for controllable, selective area unzipping of single-walled CNTs (SWNTs) into sub-5 nm graphene nanoribbons (GNRs), forming intramolecular junctions that combine GNR and SWNT in a one-dimensional (1D) nanostructure. Electrical measurements reveal a strong gate-dependent rectifying behaviour, which is intrinsic to the SWNT/GNR junction. We also investigate potential applications of these intramolecular junctions as directionally dependent field-effect transistors (FETs), logic gates and high-performance photodetectors. Unzipping of SWNTs The zero bandgap, to a certain degree, limits the applications of graphene in electronics [1] . Theoretical and experimental studies have shown that quantum confinement and edge effects can introduce a width-dependent bandgap in GNRs [9] , [10] , [11] , [12] . For electronics applications, sub-5 nm GNRs are required to exhibit semiconducting characteristics with sufficiently large bandgaps for high on/off FET operations at room temperature [9] , [10] , [11] . To date, several methods have been developed to produce GNRs, such as lithographic patterning [11] , sonication of graphite [12] or graphene sheets [13] , nanowire template etching [14] , chemical vapour deposition [15] , selective etching of graphene edges [16] , unzipping of CNTs [8] , [17] , [18] , [19] , [20] , [21] , and so on. Among them, unzipping of CNTs offers the possibility to control the morphologies of the GNRs. For example, chirality of the GNRs can in principle be determined by the diameter and chirality of the parent CNTs. This approach can benefit from progress made over the past two decades to produce CNTs in controllable length, density, alignment, diameter, and so on [8] . Although the controllability of the CNT growth has been extensively developed, the controllability of the unzipping process is still lacking. Recently, Dimiev et al . [22] presented a zinc sputtering and acid treatment route for layer-by-layer removal of graphene. Using this strategy, we developed a controllable method for unzipping SWNTs in desired areas, which can result in sub-5 nm GNRs and SWNT/GNR intramolecular junctions. SWNTs used here were produced by ethanol chemical vapour deposition on SiO 2 /Si substrates ( Supplementary Fig. S1 , experimental details in Supplementary Data ). Atomic force microscopy (AFM) characterization ( Supplementary Fig. S2 ) confirmed that most nanotubes were single-walled with diameters in the range of 1.0–2.5 nm and a mean of 1.78 nm. A small amount of nanotubes had diameters larger than 2.5 nm, and these might be attributed to double-walled nanotubes or nanotube bundles. We exposed the SWNTs to zinc sputtering, followed by dissolution in HCl aqueous solution. After this process, the mean diameter ( Supplementary Fig. S3 ) decreased to 1.24 nm, with significant portions (47.8%) with heights below 1.0 nm, indicating that some SWNTs were unzipped into single-layer GNRs. To confirm the unzipping of SWNTs, we imaged a single SWNT by AFM ( Fig. 1a ) before and after the zinc sputtering and acid treatment. The height profiles across the same location of the SWNT indicate the height decreased from 1.29 to 0.64 nm after zinc/acid treatment. The resulting GNR was continuous and uniform along its length. Except for the height, the GNR retained the general morphology of its parent nanotube, that is, its continuous filamentary structure. 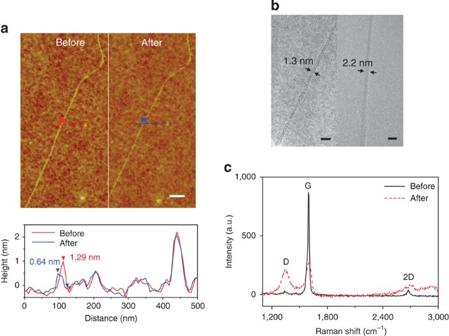Figure 1: Unzipping of SWNTs. (a) AFM images of an SWNT before (left) and after (right) unzipping. The lower figure is the height profiles across the lines in the AFM images. The arrow heads indicate the locations between which the heights were determined. Scale bar, 200 nm. (b) TEM images of an SWNT (left) and a GNR (right) transferred to the TEM grids. The scale bars are 5 nm. (c) Raman spectra measured at the same position of the sample before and after unzipping. Figure 1: Unzipping of SWNTs. ( a ) AFM images of an SWNT before (left) and after (right) unzipping. The lower figure is the height profiles across the lines in the AFM images. The arrow heads indicate the locations between which the heights were determined. Scale bar, 200 nm. ( b ) TEM images of an SWNT (left) and a GNR (right) transferred to the TEM grids. The scale bars are 5 nm. ( c ) Raman spectra measured at the same position of the sample before and after unzipping. Full size image Figure 1b shows typical transmission electron microscopy (TEM) images of an SWNT and a GNR obtained before and after zinc/acid treatment, respectively. The wall of the SWNT can be clearly distinguished, indicating a tubular structure. The GNR shows distinct topographic characteristics, a ribbon-like structure with relatively smooth edges. No wall-like structure is observed, and the width is about 2.2 nm, indicating that the product is a sub-5 nm GNR, which should have an open bandgap suitable for FET applications [9] , [10] , [11] , [12] . Figure 1c shows the typical Raman spectra measured at the same location before and after unzipping. The SWNTs display a strong G-band (1,594 cm −1 ) and a very weak D-band, indicating the high quality of the SWNTs as the starting material. After unzipping, a strong D-band (1,345 cm −1 ) and a decreased G-band (1,598 cm −1 ) were observed. The notable increase of the intensity ratio of D-band and G-band ( I D / I G ) also confirms the unzipping of SWNTs, as the decrease of G-band indicates that some carbon atoms had been removed [23] , whereas the markedly increased D-band is attributed to GNR edges and defects introduced in the unzipping process, as the edges act as defects responsible for momentum conservation in the double resonance Raman process [24] , [25] . Zinc sputtering has a key role in unzipping SWNTs. Irradiation of graphitic materials by electrons, ions, atoms, and so on, can remove carbon atoms and produce atomic size defects in the graphitic networks [26] . However, there is a threshold energy for carbon atom displacement. In the case of electron beam irradiation, the value is 18–20 eV (refs 26 , 27 ), and is 47.3 eV for Ar + ion irradiation [28] . Hahn et al . [28] , [29] found that irradiation of graphite by Ar + ion beams at 50 eV removes one surface carbon to produce an atomic size defect that did not extend further than the top layer, as this energy is only barely above the threshold for carbon displacement and the extra energy was insufficient to remove an additional carbon atom. In the case of zinc, the sputtering process can provide zinc ions with appropriate energy to permanently destroy one carbon atom layer, which as well as residual zinc can be removed in the following acid treatment, thus Dimiev et al . [22] realized layer-by-layer removal of graphene by zinc/acid treatment. Similarly, the zinc sputtering and subsequent acid treatment can remove the top exposed SWNT wall, thus unzipping SWNTs into GNRs. The detailed mechanism needs further investigation. The sputtering conditions need to be carefully controlled. As there is a threshold energy, no unzipping effect can be observed under weak sputtering conditions ( Supplementary Fig. S4 ). Controllable unzipping for intramolecular junctions Compared with other unzipping methods, the benefit of this approach is that unzipping of nanotubes can be realized in selected areas if we use poly-methyl-methacrylate (PMMA) patterns as the mask in zinc sputtering. After the process illustrated in Fig. 2 , AFM measurements ( Fig. 3a ) shows that the product coexists an SWNT with 2.09 nm height and an opened GNR with 0.64 nm height, resulting in an SWNT/GNR intramolecular junction along the SWNT at the interface. This junction configuration could be clearly distinguished in the three-dimensional (3D) AFM image ( Fig. 3b ). Figure 3c showed the height profile along the junction, revealing a continuous connexion at the interface. 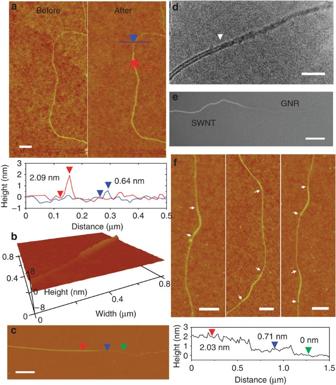Figure 3: SWNT/GNR intramolecular junctions. (a) AFM images of a SWNT before (left) and after (right) patternedly unzipping the upper part. The lower figure is the height profiles across the lines in right AFM image. A 3D AFM image (b), an AFM image (c), a TEM image (d) and an SEM image (e) of another SWNT/GNR intramolecular junctions. The right figure of (c) is the height profile along the junction. The arrow head indindicates the junction interface. (f) AFM images of the products with 2 (left), 3 (middle) and 4 (right) SWNT/GNR intramolecular junctions. The arrows indicate the positions of the junctions. The scale bars ina,c,d,eandfare 200, 500, 10 nm, 5 μm and 300 nm, respectively. The arrow heads in (a) and (c) indicate the locations between which the heights were determined. To further confirm the detailed structure, the junctions were transferred to TEM grids by PMMA. The typical TEM image, shown in Fig. 3d , reveals the junction consists of a tubular and a ribbon-like structure with a nanoscale interface between them. Figure 3e shows a typical scanning electron microscopy (SEM) image of an SWNT/GNR intramolecular junction at 1 kV acceleration voltage. We observed different contrasts at each side of the junction. The bright contrast and apparent large diameter of the SWNT at 1 kV were caused by the accumulation of electrons on SWNTs above the positively charged substrate [30] , [31] . Due to differences in electrical characteristics, a different contrast was observed in the GNR segment. Moreover, when we partly covered the SWNTs by several PMMA stripes and unzipped the uncovered segments ( Supplementary Fig. S5 ), several SWNT/GNR intramolecular junctions could be produced sequentially along the SWNTs. As an example, 2, 3 and 4 SWNT/GNR intramolecular junctions were produced along one SWNT as shown in Fig. 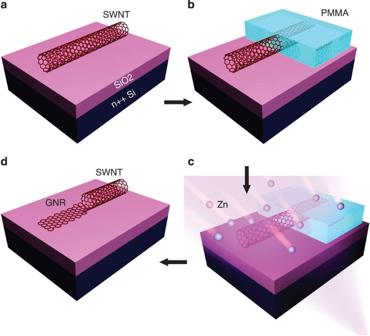3f . Figure 2: Schematic diagram of the patterned unzipping of an SWNT for producing an SWNT/GNR intramolecular junction. (a) First, an SWNT was grown on a SiO2/Si substrate. (b) PMMA was patterned on one side of the SWNT by EBL, which could protect the SWNT underneath from zinc sputtering. (c) The substrate was exposed in zinc sputtering. (d) After removing zinc and PMMA by HCl and acetone treatments, respectively, GNR was obtained at the exposed side, resulting in an SWNT/GNR intramolecular junction at the interface. (d) A schematic representation of the junction. Figure 2: Schematic diagram of the patterned unzipping of an SWNT for producing an SWNT/GNR intramolecular junction. ( a ) First, an SWNT was grown on a SiO 2 /Si substrate. ( b ) PMMA was patterned on one side of the SWNT by EBL, which could protect the SWNT underneath from zinc sputtering. ( c ) The substrate was exposed in zinc sputtering. ( d ) After removing zinc and PMMA by HCl and acetone treatments, respectively, GNR was obtained at the exposed side, resulting in an SWNT/GNR intramolecular junction at the interface. ( d ) A schematic representation of the junction. Full size image Figure 3: SWNT/GNR intramolecular junctions. ( a ) AFM images of a SWNT before (left) and after (right) patternedly unzipping the upper part. The lower figure is the height profiles across the lines in right AFM image. A 3D AFM image ( b ), an AFM image ( c ), a TEM image ( d ) and an SEM image ( e ) of another SWNT/GNR intramolecular junctions. The right figure of ( c ) is the height profile along the junction. The arrow head in d indicates the junction interface. ( f ) AFM images of the products with 2 (left), 3 (middle) and 4 (right) SWNT/GNR intramolecular junctions. The arrows indicate the positions of the junctions. The scale bars in a , c , d , e and f are 200, 500, 10 nm, 5 μm and 300 nm, respectively. The arrow heads in ( a ) and ( c ) indicate the locations between which the heights were determined. Full size image Rectification properties and related applications We fabricated electrical devices on SWNT/GNR intramolecular junctions, with four Au/Cr electrodes, a p++ Si back gate and 300 nm SiO 2 as the gate dielectric, by electron beam lithography (EBL). The device configuration is illustrated in Fig. 4a . The samples were annealed in 200 mTorr H 2 /Ar at 800 °C for 15 min before device fabrication, and to improve the contact the device was annealed in Ar at 250 °C. 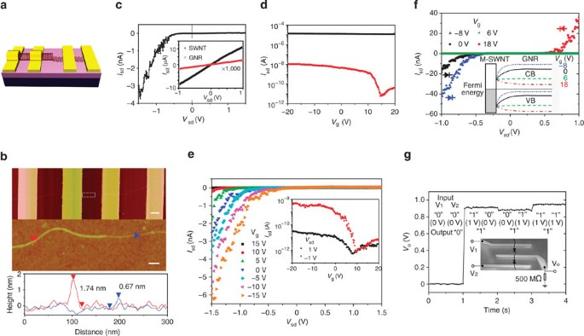Figure 4: Electrical measurement of the SWNT/GNR intramolecular junctions. (a) Bird’s-eye view of a schematic device configuration. (b) AFM image of a device with four electrodes. Scale bar, 1 μm. The middle figure is the higher magnified AFM image of the area indicated by a dashed frame, and the scale bar is 100 nm. The lower figure is the height profiles across the lines in the middle figure. The arrow heads indicate the locations between which the heights were determined. (c)Isd–Vsdcurve of the SWNT/GNR intramolecular junction. The inset isIsd−Vsdcurves of the SWNT segment (black) and the GNR segment (red). (d)Isd–Vgcurves of the SWNT segment (black) and the GNR segment (red) atVsd=−1 V. (e) Gate voltage-dependentIsd–Vsdcurves of the M–S SWNT/GNR intramolecular junction. The inset is the transfer curves of the junction atVsd=1 and −1 V, respectively. (f) Rectification behaviours of a M–S SWNT/GNR intramolecular junction in differentVgregions. The inset shows the schematic diagram of the energy band at the intramolecular junction at differentVg. (g) Output voltage of a logic OR gate for the four possible inputs: (0,0), (0,1), (1,0), (1,1) and the truth table. Inset shows schematic of the electronic circuit of the logic OR gate. (c,eandf) GNR was grounded, and a biasVsdwas applied on SWNT. Figure 4b shows AFM images of a typical device, and the enlarged image reveals the intramolecular junction is composed of a 1.74 nm diameter SWNT and a 0.67 nm high GNR. As shown in Fig. 4c , the I sd – V sd (source–drain current versus source–drain bias voltage) curves of the SWNT segment and the GNR segment are symmetrical, and the linear behaviour of the curves indicates an Ohmic contact with the Au/Cr electrodes. The GNR segment has a lower conductivity by three to four orders of magnitude compared with the SWNT segment, which is attributed to the opened bandgap, edge scattering and local-defect scattering in the ultra-narrow conducting channel [8] , [11] , [17] , [32] . In contrast, the I sd – V sd characteristic across the junction is highly nonlinear and asymmetric with rectification ratio (RR=current at −1.5 V/current at +1.5 V) of ~160, resembling that of a rectifying diode with a turn-on voltage ( V T ) at about −0.5 V. For a further understanding of the rectification behaviour, we measured the transfer curves of both the SWNT segment and the GNR segment ( Fig. 4d ). Different gate-voltage ( V g )-dependent behaviours ( Supplementary Figs S6 and S7 ) of I sd were observed. The poor V g dependence of the SWNT segment is indicative of its metallic nature, whereas the GNR segment shows a typical p-type semiconducting behaviour, affording FETs with an on/off ratio of ~10 3 at V sd =−1 V. The semiconducting nature of the GNR originates from the bandgap generated by its nanoscale width [9] , [10] , [11] , [12] , and the p-type behaviour is attributed to absorption of oxygen or water in air, similar to the CNT FETs in air [33] . The mobility of the GNR was about 19.7 cm 2 V −1 s −1 , and the relatively low mobility is attributed to edge defects and local defects introduced in the unzipping process, which could act as the carrier scattering centres in the ultra-narrow conducting channel [34] . Therefore, at the interface of the metallic SWNT and the semiconducing GNR, a metal–semiconductor (M–S) junction is formed, which should be responsible for the diode-like rectifying behavior [35] . Theoretical simulations (see details in Supplementary Information ) also reveal the gate-dependent rectifying behaviour across the junction ( Supplementary Figs S8–S12 ). Figure 4: Electrical measurement of the SWNT/GNR intramolecular junctions. ( a ) Bird’s-eye view of a schematic device configuration. ( b ) AFM image of a device with four electrodes. Scale bar, 1 μm. The middle figure is the higher magnified AFM image of the area indicated by a dashed frame, and the scale bar is 100 nm. The lower figure is the height profiles across the lines in the middle figure. The arrow heads indicate the locations between which the heights were determined. ( c ) I sd – V sd curve of the SWNT/GNR intramolecular junction. The inset is I sd − V sd curves of the SWNT segment (black) and the GNR segment (red). ( d ) I sd – V g curves of the SWNT segment (black) and the GNR segment (red) at V sd =−1 V. ( e ) Gate voltage-dependent I sd – V sd curves of the M–S SWNT/GNR intramolecular junction. The inset is the transfer curves of the junction at V sd =1 and −1 V, respectively. ( f ) Rectification behaviours of a M–S SWNT/GNR intramolecular junction in different V g regions. The inset shows the schematic diagram of the energy band at the intramolecular junction at different V g . ( g ) Output voltage of a logic OR gate for the four possible inputs: (0,0), (0,1), (1,0), (1,1) and the truth table. Inset shows schematic of the electronic circuit of the logic OR gate. ( c , e and f ) GNR was grounded, and a bias V sd was applied on SWNT. Full size image We also measured the I sd – V sd characteristics of the M–S SWNT/GNR junction for different V g ( Fig. 4e ), which resembles that of a directionally dependent FET with a current under forward bias about two orders of magnitude larger than that under reverse bias. The on/off ratio of the device was about 10 4 under forward bias, and decreased to about 10 2 under reverse bias. By applying a negative V g , the I sd – V sd curves became increasingly asymmetric, and RR increased to ~400 at V g =−15 V. It is interesting that the V T shifted as a function of V g , and a positive shift of about 1.2 V was observed when V g varied from 10 to −15 V. Besides M–S junctions, we also observed semiconductor–semiconductor (S–S) SWNT/GNR intramolecular junctions. Similar to M–S junction, S–S junction also exhibited a gate-dependent rectifying behaviour ( Supplementary Fig. S13 ), however, the rectifying behaviour varied with each S–S junction, and some had a very small RR (<5, Supplementary Fig. S14 ). The different rectifying behaviour of each S–S junction is attributed to the barrier formed between semiconductors with different band structures, in good agreement with the theoretical simulation ( Supplementary Figs S8, S9 and S15 ). To improve the performance of the GNR and junction devices, we further annealed the samples in 100 mTorr pure H 2 at 1,000 °C for 40 min before device fabrication. An improved mobility of GNRs was observed, ranging from ~29 to 120 cm 2 V −1 s −1 , with a reduced resistance. RR (at ±1.0 V) of the M–S junction device increased to the range of 10 −3 to 10 −4 . For instance, RR is 3.5 × 10 3 at V g =0 in Fig. 4f and Supplementary Fig. S16a . A strong V g dependence of the rectifying behaviour was observed ( Fig. 4f and Supplementary Fig. S16b ), and the rectifying curves can be categorized as three types (i, ii, iii) at different V g regions. When V g =6 V, the device was depleted in an insulative state (ii). When V g <6 V or >6 V, we observed a forward (i) or a reverse (iii) rectifying behaviour, and a field-effect behaviour which resembles that of a forward (i) or a reverse (iii) directionally dependent FET, respectively. The inset of Fig. 4f shows a proposed energy diagram across the M-SWNT/GNR junction. Due to the p-type doping of GNR in air, the conductive band and the valence band bend upward, forming a ‘downward’ potential barrier (for holes). The barrier structure can be significantly modulated by a gate electric field. With a negative V g , holes are accumulated in GNR, resulting in thinning the hole barrier and increasing the hole density, thus current increases under forward bias, corresponding to that of a forward directionally dependent FET (i). However, with a positive V g , the energy band bends downward, resulting in decreasing of the carrier (hole) density and widening of the barrier. When positive V g increases to a certain value, the GNRs can be fully depleted into an insulative state with a flat band structure (ii). Further increasing the positive V g will cause n-type (electron) doping of GNR, where electrons become the majority carrier in the channel and the band-bending direction changes. As a result, a barrier for electrons forms, which results in a reverse rectifying behaviour and a reverse directionally dependent FET behaviour (iii). To demonstrate a logic application, an OR gate was constructed from two SWNT/GNR intramolecular junctions along a nanotube. Figure 4g shows the schematic and the input–output voltage response of this device. The output is a logic 0 only when both inputs are a logical 0 (0 V), as neither junctions is forward biased. When either or both of the inputs are a logical 1 (1 V), at least one junction is conducting and the output ( V o ) will be logic 1. Photoconducting properties and related applications One significant potential application of graphene and CNTs is in optoelectronics [36] . Our SWNT/GNR intramolecular junctions provide us a model system to realize optoelectronics in an all-carbon nano-system. 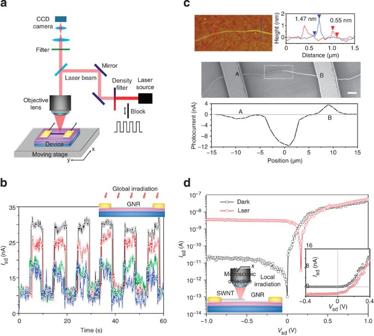Figure 5: Photoconducting properties of the GNR and the intramolecular junction. (a) Schematic description of the experimental setup of the photoelectric measurement. (b) Photoconductivity response of a GNR atVsd=0.5 V when a global laser beam with PI at 13.2 (black), 9.6 (red), 6.4 (green) and 4.5 (blue) kW cm−2is turned on and off. (c) An SEM image of a SWNT/GNR junction device. Scale bar, 2 μm. The upper insets are an AFM image of the area indicated by a dash frame in the SEM image, and the height profiles across the lines in the AFM image. The arrow heads indicate the locations between which the heights were determined. The lower inset showsIpatVsd=0 V when a 2-μm-size focused laser beam scans along the junction from A to B as marked in the SEM image. (d)Isd–Vsdcurves of the SWNT/GNR junction device in dark (black) and when a 34.7 kW cm−2laser beam was focused at the junction (red). The right inset is theIsd–Vsdcurves with linearY-axis, and the left inset depicts the experiment setup. (c,d) SWNT was grounded,Vsd,IporVpwere applied or measured on GNR. CCD, charge-coupled device. Figure 5a shows the schematic of our photocurrent measurement system. Objective lenses with the magnification X5 or X50 were used to focus a laser beam (wavelength 660 nm) into a 20 or 2 μm spot for global or local irradiation of the device, respectively. An obvious photoconductivity response was detected, when a 20-μm-size laser beam was focused globally on the whole GNR device at V sd =0.5 V ( Fig. 5b ). The conductivity increased about three times using a laser with power intensity (PI) at 13.2 kW cm −2 . Both a perfect on/off photoconductivity response and a PI-dependent photoconductivity were observed, confirming the semiconducting behaviour of GNRs. Figure 5: Photoconducting properties of the GNR and the intramolecular junction. ( a ) Schematic description of the experimental setup of the photoelectric measurement. ( b ) Photoconductivity response of a GNR at V sd =0.5 V when a global laser beam with PI at 13.2 (black), 9.6 (red), 6.4 (green) and 4.5 (blue) kW cm −2 is turned on and off. ( c ) An SEM image of a SWNT/GNR junction device. Scale bar, 2 μm. The upper insets are an AFM image of the area indicated by a dash frame in the SEM image, and the height profiles across the lines in the AFM image. The arrow heads indicate the locations between which the heights were determined. The lower inset shows I p at V sd =0 V when a 2-μm-size focused laser beam scans along the junction from A to B as marked in the SEM image. ( d ) I sd – V sd curves of the SWNT/GNR junction device in dark (black) and when a 34.7 kW cm −2 laser beam was focused at the junction (red). The right inset is the I sd – V sd curves with linear Y -axis, and the left inset depicts the experiment setup. ( c , d ) SWNT was grounded, V sd , I p or V p were applied or measured on GNR. CCD, charge-coupled device. Full size image More interestingly, the M–S SWNT/GNR devices showed excellent photoconductive properties. As shown in the SEM and the enlarged AFM images ( Fig. 5c ), the junction was composed of a 1.47 nm height SWNT and a 0.55 nm height GNR. The I – V curve in dark ( Fig. 5d ) shows a typical rectifying behaviour with RR ( V sd =±1 V) about 2.2 × 10 3 . Under global irradiation, a photocurrent ( I p ) response of the junction device ( Fig. 6a ) was detected up to –75 pA at V sd =0 V at PI=96.3 W cm −2 , whereas no obvious photocurrent was detected when the laser was focused globally on the GNR or SWNT device ( Supplementary Fig. S17 ), which suggests that the photocurrent originates from the junction. To confirm this, a 2-μm-size focused laser beam with PI=98.6 kW cm −2 was utilized, and I p generated by local irradiation over each point was recorded when the laser spot was scanned between two electrodes across the junction at V sd =0 V ( Fig. 5c ). The largest I p (–11.6 nA) was observed at the junction, whereas a negative I p (–1.57 nA) and a positive I p (3.66 nA) were detected near the electrode/GNR interface and SWNT/electrode interface, respectively. Under local irradiation (PI=34.7 kW cm −2 ) at the junction, the I sd – V sd curve ( Fig. 5d ) yielded an open-circuit voltage of 0.17 V, and a short-circuit current of –2.9 nA. The reverse current increased more than two orders, whereas the current increased only a little under forward bias. 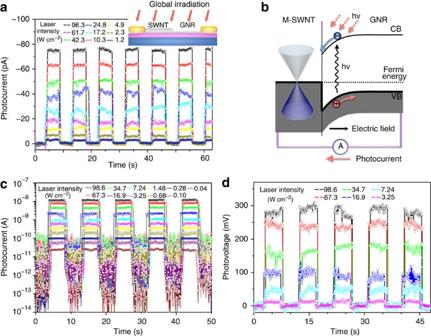Figure 6: Photoconducting response of the intramolecular junction. (a)Ipresponse of the SWNT/GNR junction (atVsd=0 V) when the global laser beam is switched on and off. (b) Schematic band diagram at the junction under irradiation. (c,d)Ip(atVsd=0 V) andVp(atIsd=0 A) response when the laser beam focused on the SWNT/GNR junction was switched on and off. (a,candd) SWNT was grounded,Vsd,IporVpwere applied or measured on GNR. CB, conductive band. Figure 6: Photoconducting response of the intramolecular junction. ( a ) I p response of the SWNT/GNR junction (at V sd =0 V) when the global laser beam is switched on and off. ( b ) Schematic band diagram at the junction under irradiation. ( c , d ) I p (at V sd =0 V) and V p (at I sd =0 A) response when the laser beam focused on the SWNT/GNR junction was switched on and off. ( a , c and d ) SWNT was grounded, V sd , I p or V p were applied or measured on GNR. CB, conductive band. Full size image The remarkable photo-response is attributed to the photo-generated electron-hole pairs. In the case of the GNR device, a potential drop maintained by the applied bias results in an external electric field along the GNR, which separates the excited electron-hole pairs and gives rise to a conductivity response to the laser irradiation ( Supplementary Fig. S18 ). In the case of the M–S GNR/SWNT junction, the presence of band bending at the junction results in a strong local electric field, which separates the electron-hole pairs. The holes move towards the GNR, and the photo-generated electrons diffuse to the SWNT, leading to a reverse I p at V sd =0 V and a forward photovoltage ( V p ) under open circuit ( Fig. 6b ). As a result, orders of magnitude increase of the reverse current was observed under irradiation because of the reverse I p . Due to the different band-bending directions at the electrode/GNR (or SWNT) and GNR (or SWNT)/electrode interface, opposite I p were generated at both interfaces, which causes an invisible photocurrent response of the GNR (or SWNT) device under global irradiation [37] , [38] , [39] , [40] . Owing to the asymmetric configuration, GNR/SWNT devices show a considerable photocurrent response under global irradiation. More importantly, excitons are expected to form in the bulk sections of the 1D structure because of strong 2D quantum confinement, and thus a much enhanced Coulombic electron-hole coupling was observed in the cross-section. Consequently, the optical absorption probability, the drift-diffusion velocity of the carriers, and the carrier relaxation time notably increases [37] , [41] , [42] , [43] , [44] . These, as well as the high efficiency for electron-hole separation at the SWNT/GNR junction, give rise to a strong photo-response. An impressive I p up to −11.6 nA ( V sd =0 V) and a V p up to 270 mV were achieved under local irradiation with PI=98.6 kW cm −2 . The external photoresponsivity was about 3 mA W −1 , which was even larger than that of the 2D graphene (1.5 mA W −1 at V sd =0, 632.8 nm laser) [39] , p–n junctions of 2D graphene (1 mA W −1 , 632.8 nm laser) [38] , or nanotubes ( I p =1 nA when PI=100 kW cm −2 , 781 nm laser) [40] . I p ( Fig. 6c , Supplementary Fig. S19 ) and V p ( Fig. 6d ) depend linearly and logarithmically, respectively, on the PI, consistent with the systematic increase in photo-generated carriers [45] . Owing to both the high sensitivity and the excellent PI-dependent photoconductive properties, the SWNT/GNR intramolecular junctions have potential applications as high-performance photodetectors. In this article, we unzipped SWNTs into sub-5 nm GNRs by the zinc/acid sputter-etching method. The resulting GNRs exhibited typical semiconducting behaviour, which could address the problem of the extreme chirality dependence of metal or semiconductor nanotubes and zero bandgap pristine graphene in future electronics. More importantly, compared with other unzipping routes, the benefit of this approach is that the unzipping can be realized in selected areas, resulting in SWNT/GNR intramolecular junctions along the nanotubes. Electrical studies showed a gate-dependent rectifying behaviour across these junctions, which is intrinsic to the SWNT/GNR junction, in agreement with the theoretical simulations. Moreover, we demonstrated prototype applications in directionally dependent FETs, logic gates and photodetectors. An impressive photocurrent as high as −11.6 nA and a photovoltage up to 270 mV were achieved, indicating their potential applications in high-performance photodetectors or even in nano-electronic power sources. We believe this work is valuable for both the scientific understanding and practical applications of GNRs, and graphene-based junctions in electronics and optoelectronics. Preparation of GNRs SWNTs were synthesized on Si substrates with 300-nm oxidation layer by chemical vapour deposition using FeCl3 (Sigma-Aldrich) as the catalyst and ethanol as the carbon source. Next, PMMA (5% 950K PMMA in Anisole) was spin coated on the substrates, and then was patterned by EBL. The patterned substrate was then exposed to zinc sputtering (Denton Vacuum Discovery-18 sputtering system, 50 W RF, 2 min, in 100 sccm Ar, experimental details in Supplementary Information ). After that, the zinc was dissolved by immersing the substrates in 0.1 M HCl solution for 5 min, and then the substrate was washed in distilled water several times and air dried. PMMA was removed in acetone vapour. Finally, to improve the quality of the samples, the SiO 2 /Si substrates were annealed in H 2 /Ar (20% H 2 ) gas at 800 °C for 15 min at a pressure of 200 mTorr. Characterization of GNRs The samples were measured by AFM (Veeco D3000, tapping mode), Raman (Renishaw 2000, 514 nm), field emission SEM (JEOL JSM-6700F, acceleration voltage: 1 kV) and field emission TEM (JEOL 2010F, acceleration voltage: 200 kV). To prepare the TEM sample, GNRs, SWNTs or junctions were transferred from the SiO 2 /Si substrate to TEM grids by PMMA, and then the PMMA was removed by acetone vapour, and the sample was annealed at 300 °C for 20 min in Ar (purity: 99.999%) at a pressure of 200 mTorr. Device fabrication and electrical measurement First, we imaged the substrate by SEM to locate the sample (1 kV and 5 μA were used to avoid the destruction by electron beam) after thermal annealing. The source–drain electrodes (5/30 nm Cr/Au) were then patterned on the sample by EBL and electron beam deposition. To obtain a better contact between the sample and the Au/Cr electrodes, thermal annealing was performed in an Ar atmosphere at 250 °C for 15 min using a tube furnace. For electrical measurement, both the Cr/Au electrodes and the p++ Si back gate were wire bonded using Al wires, and the electrical characterization was carried out in air at room temperature by a semiconductor analyser (Keithley 2636A). Photoconductivity measurement Two approaches were implemented: a globally approach where the laser was directly irradiated as a broad beam or was focused as 20-μm-size spot on the whole device, and a local approach where the laser was focused to a 2-μm-size spot on different sections of the device. The PI of the laser (660 nm, PhotoniTech Pte. Ltd.) was controlled by density filter and was measured by a laser power metre. The electrodes were wire bonded out, the I p and V p were measured by semiconductor analyser (Keithley 6430) in air at room temperature. How to cite this article: Wei, D. et al . Controllable unzipping for intramolecular junctions of graphene nanoribbons and single-walled carbon nanotubes. Nat. Commun. 4:1374 doi: 10.1038/ncomms2366 (2013).